Host–parasite network structure is associated with community-level immunogenetic diversity Genes of the major histocompatibility complex (MHC) encode proteins that recognize foreign antigens and are thus crucial for immune response. In a population of a single host species, parasite-mediated selection drives MHC allelic diversity. However, in a community-wide context, species interactions may modulate selection regimes because the prevalence of a given parasite in a given host may depend on its prevalence in other hosts. By combining network analysis with immunogenetics, we show that host species infected by similar parasites harbour similar alleles with similar frequencies. We further show, using a Bayesian approach, that the probability of mutual occurrence of a functional allele and a parasite in a given host individual is nonrandom and depends on other host–parasite interactions, driving co-evolution within subgroups of parasite species and functional alleles. Therefore, indirect effects among hosts and parasites can shape host MHC diversity, scaling it from the population to the community level. Species interactions are a source of selective pressures that can maintain genetic variability in host populations, parasitism being a classic example [1] , [2] , [3] . In particular, this is true for the major histocompatibility complex (MHC) in vertebrates. The MHC is a highly polymorphic region in the genome comprising closely linked genes. These genes encode cell-surface glycoproteins that recognize and present foreign antigens, such as those of invading parasites, to T lymphocytes thereby initiating an immune response [4] . Thus, at the host individual level, certain MHC alleles confer resistance/susceptibility to some parasites but not to others [5] , [6] , [7] . Parasite-mediated selection drives MHC polymorphism at the host population level because of the evolutionary interplay between parasites and MHC-encoded proteins within a host individual [8] , [9] . Indeed, several studies have shown that in a host population, parasite diversity—the number and identity of parasite species and their abundance in a host population—is correlated with MHC diversity—the number of MHC alleles in a host and their identity—but not with genetic diversity assessed with neutral markers such as microsatellites or mitochondrial genes [5] , [10] . At the species level, studies of host interspecific variation in MHC are scarce but have confirmed a positive correlation between parasite species richness and MHC richness across species [11] , [12] . However, these studies were based on data collected from the literature, dealt with host species that were not simultaneously surveyed both for parasites and MHC alleles, and did not consider the functional diversity of alleles. More importantly, the way interactions among hosts and parasites are distributed was ignored and thus no study examined the association between multiple host and parasite interactions and MHC diversity. Although few studies have explored the effects of multiple parasites on MHC diversity [7] , [10] , [13] , they were conducted within a population of a single host. Interactions between multiple hosts and parasites are often depicted as a host–parasite network. Considering network structure is crucial because, in nature, species do not live in isolation but rather belong to a community where species affect each other directly or indirectly [14] , [15] . In this community-wide context, the prevalence of a given parasite species in a given host species may depend on its prevalence in other host species in the community. Therefore, the selective pressure exerted by the parasite may be influenced by indirect species interactions and may itself influence diversity of MHC alleles directly involved in the host-parasite interaction ( Fig. 1 ). That is, the structure of the host–parasite network may correlate with MHC diversity among host species. Using a unique data set on a community of rodents, their helminths parasites and their MHC alleles, we tackle here, for the first time, this largely unexplored research topic by integrating complex network theory with immunogenetics. 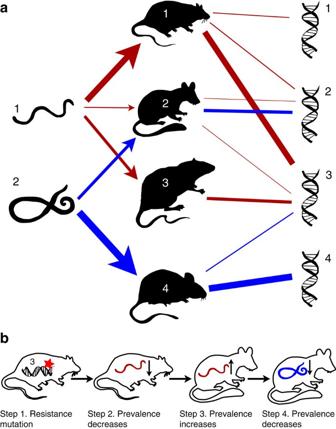Figure 1: An example for the interplay between host–parasite and host–supertype networks. (a) On the left, host–parasite interactions between helminths and rodent species (ecological network). Arrow width is proportional to the prevalence of a given parasite on a host. On the right, the immunogenetic host-supertype network in which interactions represent the frequencies (indicated by line width) of supertypes harboured by individuals of a given host that are infected by each parasite (indicated by different colours). (b) A theoretical example showing how in a community-wide context, species and MHC supertypes affect each other indirectly with possible cascading indirect effects. Imagine that a mutation for resistance (depicted by a red star) occurs in an allele from supertype no. 3 in the population of host no. 1 (step 1), causing the prevalence of parasite no. 1 to decrease in that host (step 2). Parasite no. 1 now switches to host no. 2 (step 3), thus reducing the prevalence of parasite no. 2 in host no. 2 due to competition (step 4). Figure 1: An example for the interplay between host–parasite and host–supertype networks. ( a ) On the left, host–parasite interactions between helminths and rodent species (ecological network). Arrow width is proportional to the prevalence of a given parasite on a host. On the right, the immunogenetic host-supertype network in which interactions represent the frequencies (indicated by line width) of supertypes harboured by individuals of a given host that are infected by each parasite (indicated by different colours). ( b ) A theoretical example showing how in a community-wide context, species and MHC supertypes affect each other indirectly with possible cascading indirect effects. Imagine that a mutation for resistance (depicted by a red star) occurs in an allele from supertype no. 3 in the population of host no. 1 (step 1), causing the prevalence of parasite no. 1 to decrease in that host (step 2). Parasite no. 1 now switches to host no. 2 (step 3), thus reducing the prevalence of parasite no. 2 in host no. 2 due to competition (step 4). Full size image We show that host species infected by similar parasites harbour similar MHC functional alleles with similar frequencies after controlling for phylogenetic effects. Also, the indirect effects among hosts and parasites influence the probability of mutual occurrence of a functional MHC allele and a parasite in a given host individual. Therefore, the ecology of host–parasite interactions and the evolution of MHC are intertwined, and indirect effects among hosts and parasites can shape host MHC diversity, scaling it from the population to the community level. Data set An extensive helminth survey was conducted in six localities in southeast Asia ( Supplementary Fig. 1 ) on 950 specimens of 11 murinae rodent species within the framework of the Community of Rodents and their Pathogens project ( www.ceropath.org ) [16] . Of these, 440 individuals were parasitized by 26 helminth taxa (22 identified to species level and 4 to family level) ( Supplementary Tables 1–3 ). Infection usually depends on species co-occurrence in space and time. Also, hosts of the same species but from different populations may be exposed to different selective pressures, thereby creating variation in MHC due to local adaptation. We therefore first analysed data using rodent individuals captured in a single locality (Loei). Despite geographical distance between the localities, they all belong to the same Indochina bioregion and are rather homogeneous in their environmental conditions [17] . Furthermore, all rodent species from other localities occurred in Loei ( Supplementary Table 1 ). Therefore, we pooled data from the six localities and considered rodents as belonging to a single community to increase statistical power. This did not change our results qualitatively (see below) and we thus focus on the results of analyses done on pooled data. Each individual rodent was genotyped using a portion of the MHC class II DRB exon-2 functional gene that recognizes extracellular parasites such as helminths [18] . Foreign antigens are recognized by particular amino acids of the MHC molecule called the antigen-binding site. Some MHC alleles code for MHC molecules that bind an overlapping gamma of peptides. This happens when the antigen-binding sites of the coded molecules possess amino-acid sequences with similar physical and biochemical properties. Such alleles are thus functionally similar and can be classified into supertypes based on their antigen-binding site amino-acid sequences [19] , [20] , [21] . Because we were interested in functional diversity, and to avoid sparse networks caused by an excess of alleles with very few interactions, we first clustered functionally similar alleles into supertypes following refs 22 , 23 (see Methods section and Supplementary Fig. 2 ). This resulted in 24 supertypes but we omitted from statistical analysis one supertype (no. 23) that was not harboured by any infected individual, and thus 23 supertypes remained for analysis. Host–parasite and host–supertype networks are correlated We constructed a host–parasite ‘ecological network’ and a host–supertype ‘immunogenetic network’ in which the value of interactions were set as parasite prevalence or supertype frequency, respectively (matrix cell values in Fig. 2 ). If parasite-mediated selection is associated with the structure of the host–parasite network, then there should be a correlation between the identity and prevalence of parasite species and the identity and frequency of supertypes that hosts are infected by or harbour, respectively. Yet, since host species share a common evolutionary history, we have to account for the role that host phylogeny plays in the distribution of supertypes among host species ( Fig. 2 ). We applied a partial Mantel’s test to quantitative dissimilarity matrices based on the ecological and immunogenetic networks, while using a matrix of pairwise phylogenetic distances to control for phylogenetic effects [24] , and found a positive and significant correlation between the host–parasite and host–supertype matrices ( r =0.62, P =0.001; Supplementary Fig. 3 ). This means that two host species, infected by similar parasite species with a similar prevalence, tend to harbour the same MHC supertypes with similar frequencies. These results were robust to host abundances, to the number of parasites that infect a host, to taxonomic resolution of parasite species, to different phylogenetic trees and to statistical ‘group effects’ ( Supplementary Methods ). 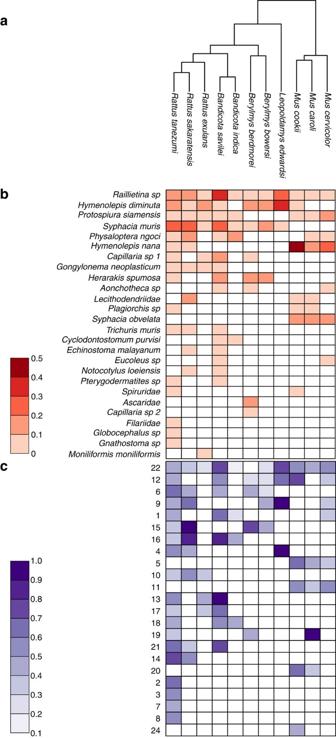Figure 2: Host phylogeny and the host–parasite and host-supertype matrices. (a) Host phylogeny. An ultrametric tree is presented for convenience. (b) Parasite prevalence: the fraction of individuals of a given host species (columns) infected by a given parasite (rows). Rows are sorted from the most generalist parasite to the most specialist one. (c) MHC supertype frequency: number of infected individuals of a given host species (columns) with a given supertype (rows), divided by the total number of individuals of that host harbouring that supertype. One supertype (no. 23) was not considered as it was not harboured by any infected individuals. Rows are sorted from the most widely distributed supertype among hosts to the most species-specific. Figure 2: Host phylogeny and the host–parasite and host-supertype matrices. ( a ) Host phylogeny. An ultrametric tree is presented for convenience. ( b ) Parasite prevalence: the fraction of individuals of a given host species (columns) infected by a given parasite (rows). Rows are sorted from the most generalist parasite to the most specialist one. ( c ) MHC supertype frequency: number of infected individuals of a given host species (columns) with a given supertype (rows), divided by the total number of individuals of that host harbouring that supertype. One supertype (no. 23) was not considered as it was not harboured by any infected individuals. Rows are sorted from the most widely distributed supertype among hosts to the most species-specific. Full size image Parasite–supertype associations across hosts are nonrandom We further explored this first evidence using a Bayesian approach that quantified parasite–supertype associations across host species ( Fig. 3 ). This analysis estimates the probability of an individual host infected by a given parasite species to harbour a given supertype. This probability can be interpreted as a proxy for the resistance/susceptibility that a given supertype provides against a given parasite as compared with all other supertypes across hosts. A high probability means that in hosts where the parasite occurs, the supertype also occurs with high probability, and thus individuals harbouring that supertype are susceptible to the parasite. The advantage of this approach is threefold. First, we represent the same data in a different way, and obtaining similar results will strengthen our conclusions. Second, we can gain a new insight into our system: the probability of obtaining a given supertype s k given a parasite p j , calculated across hosts (see Fig. 3 and Methods section). Third, the calculation of the probability of a given parasite–supertype association is based on all host–parasite interactions, thus considering the structure of the host–parasite network. 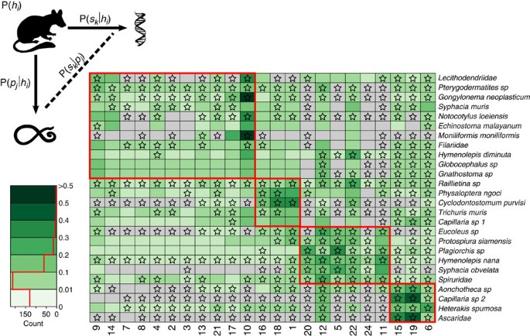Figure 3: Parasite-supertype association matrix. Matrix values depict the probability of sampling an individual of any host species infected by parasite speciespjthat harbours supertypesk—P(sk|pj). This probability of association is a proxy for the resistance a given supertype provides against a given parasite regardless of the identity of the host species, with higher probabilities indicating lower resistance. This is indicated by the green shades in the legend (the darker the shade of green colour the lower the resistance). The histogram in the legend (red line) depicts the distribution of association values. Grey cells indicate that the supertype and parasite did not co-occur in any host. Stars indicate statistically significant differences of the observed parasite-supertype probabilistic associations from random when compared with 1,000 reshuffled matrices. Modules of supertypes and parasites indicate subgroups with higher potential to co-evolve and are marked with a red border. The matrix was calculated using a Bayesian network with three nodes: host species, parasite species and MHC supertype, by combining the following conditional probabilities: probability of sampling a parasite speciespjon a given host specieshi, P(pj|hi), the probability of sampling a supertypeskon a host specieshi, P(sk|hi) and the probability of obtaining a host P(hi). Figure 3: Parasite-supertype association matrix. Matrix values depict the probability of sampling an individual of any host species infected by parasite species p j that harbours supertype s k —P( s k | p j ). This probability of association is a proxy for the resistance a given supertype provides against a given parasite regardless of the identity of the host species, with higher probabilities indicating lower resistance. This is indicated by the green shades in the legend (the darker the shade of green colour the lower the resistance). The histogram in the legend (red line) depicts the distribution of association values. Grey cells indicate that the supertype and parasite did not co-occur in any host. Stars indicate statistically significant differences of the observed parasite-supertype probabilistic associations from random when compared with 1,000 reshuffled matrices. Modules of supertypes and parasites indicate subgroups with higher potential to co-evolve and are marked with a red border. The matrix was calculated using a Bayesian network with three nodes: host species, parasite species and MHC supertype, by combining the following conditional probabilities: probability of sampling a parasite species p j on a given host species h i , P( p j | h i ), the probability of sampling a supertype s k on a host species h i , P( s k | h i ) and the probability of obtaining a host P( h i ). Full size image The resulting parasite–supertype network ( Fig. 3 ) contained all 23 supertypes and 26 parasites, with connectance (proportion of realized interactions out of all possible ones) of 72%, indicating that 28% of the potential supertype and helminths associations were not realized in any host. The values of the probabilistic associations were not affected by host abundance ( Supplementary Methods ). The first important result evident from this analysis is that the association between supertypes and parasites is variable across the host community: Whereas the association of some parasites to supertypes is homogeneous for all supertypes, other parasites are strongly associated with specific supertypes. For instance, hosts are susceptible to Syphacia muris to a similar extent, regardless of the supertypes they harbour but hosts that harbour supertype no. 10 are more susceptible to Moniliformis moniliformis than others. Similarly, the resistance some supertypes (for example, supertypes no. 7 and no. 8) provide is homogeneous to all parasites, whereas others (for example, supertypes no. 10 and no. 19) do not confer resistance to specific parasites. This analysis constitutes the first across-species analysis of the associations between multiple hosts, parasites and supertypes, and indicates that the diversity of MHC supertypes across hosts is associated with the structure of the host–parasite network. To further examine whether the observed parasite–supertype probabilistic associations are correlated with the structure of the host–parasite network, we compared the parasite–supertype matrix ( Fig. 3 ) to 1,000 matrices recalculated after reshuffling the host–parasite interactions ( M rand ). If the observed associations between parasites and supertypes ( M obs ) are not correlated with the host–parasite network structure, then they are determined by a random process and should resemble the values obtained in the random matrices. We compared cell values of M obs with distributions of their respective cell values from M rand obtained by two null models that reshuffle only the values or the values and structure of the host–parasite matrix. We found that 47% and 55% of the associations, respectively, significantly differed from random ( P <0.05; two-tailed permutation tests), accounting for 66% of the parasite–supertype associations for the two null models combined ( Fig. 3 and Supplementary Figs 4–6 ). These results were robust to host abundance and parasite taxonomic resolution ( Supplementary Methods ). This provided a second strong evidence for the interplay between host–parasite network structure and the diversity of MHC in different hosts. Networks are nested If indeed there is an interplay between the ecological and immunogenetic networks, then we should be able to predict a structural property of the immunogenetic host–supertype network based on the ecological host–parasite network. One common structural property of ecological networks is nestedness. In a nested host–parasite network, hosts infected by few parasite species (further referred to as ‘specialist’ hosts) tend to be parasitized by complete subsets of the parasites that infect more ‘generalist’ hosts—a common pattern in ecological networks [25] , [26] . The structure of the host–parasite network studied here was significantly nested (NODF=51.8, P <0.001; ref. 27 ). Thus, a substantial proportion of interactions exists among a ‘core’ of generalist hosts and parasites, which are probably those most associated with the diversity of MHC. This finding leads us to predict that hosts with low MHC richness (that harbour few supertypes) will harbour subsets of the supertypes harboured by MHC-rich hosts, resulting in a nested host-supertype network. This prediction was confirmed (NODF=50.3, P <0.001). The nested structure is of particular interest because parasite species differ in their host specificity. Thus, parasites specific to one or few hosts may encounter only a limited spectrum of supertypes. Hence, we can predict a nested structure in the parasite–supertype network because, owing to the nested structure of the host–parasite network, parasites infecting subsets of the hosts that more generalist parasites infect should also encounter subsets of supertypes harboured by those hosts. This prediction was also confirmed (NODF=78.7, P <0.001). However, nestedness is a qualitative measure that ignores parasite identity. We can further predict that if specificity is driving the observed patterns, then generalist parasites (infecting multiple hosts) will also be associated with many supertypes. If no such correlation is found, then parasite specificity is not a major factor to consider in our system. An additional analysis of parasite specificity that considered the quantitative nature of the networks and parasite identity showed that parasites specific to particular hosts are not necessarily specific to particular supertypes (Pearson’s correlation; r =0.2, P =0.34; Supplementary Fig. 7 ). This happens because some parasites with high host specificity infect hosts with high MHC diversity (for example, Gnathostoma sp. is specific to Rattus tanezumi that harbours many supertypes; Fig. 2 ). Taken together, these two analyses of specificity suggest that the interplay between the ecological and immunogenetic networks is not driven by patterns of parasite specificity, but that there is a predictable nested pattern in the selection regime between parasites and supertypes, mediated through hosts. Parasite–supertype co-evolution From an evolutionary perspective, the molecular affinity between the proteins coded by given supertypes and parasites should lead to tight associations between subgroups of parasites and supertypes in our network. We examined this hypothesis using modularity analysis and found that the parasite–supertype network had four modules ( Fig. 3 ). Supertypes and parasites within the same module interact with each other to a greater extent than with supertypes or parasites from other modules, suggesting a higher potential of parasite–supertype coevolution. The modularity of the observed parasite–supertype association network ( Q =0.37) was significantly higher than that of random networks assembled as above using both null models ( P <0.001 for both null models), indicating that the modular structure represented true co-evolutionary interactions rather than random associations between hosts and parasites. Analysis of a single community In Loei, there were 342 rodent individuals (abundance ranged between 8 and 84; Supplementary Table 1 ) belonging to 11 species. These species were parasitized by 18 of the 26 helminths taxa (70%) in the pooled data set. There was a positive and significant correlation between the two host–parasite and host–supertype matrices, after controlling for phylogenetic effects ( r =0.7, P =0.001). This correlation was maintained when controlling for host abundances and statistical ‘group effects’ ( Supplementary Methods ). The parasite–supertype matrix contained all 18 helminths taxa and 17 supertypes. The connectance of this network was 65%. When compared with the two null models that reshuffle only the values or the values and structure of the host–parasite matrix, we found that 39% and 58% of the associations, respectively, significantly differed from random ( P <0.05; two-tailed permutation tests), accounting for 67% of the parasite–supertype associations for the two null models combined. The modularity of the observed parasite–supertype association network ( Q =0.37) was significantly higher than that of random networks ( N =1,000) assembled as beforehand using the two null models that shuffle interaction values or values and network structure ( P <0.001 for both). The network had three modules. The host–parasite, host–supertype and parasite–supertype networks were all significantly nested (NODF=48.4, 44.4 and 80.8, P <0.01 for all three networks). As with the pooled data, parasites specific to particular hosts were not specific to particular supertypes (Pearson’s correlation; r =0.37, P =0.13). This study is the first to consider the structure of the associations between multiple parasites and hosts in the context of functional MHC diversity, leading to novel insights regarding the ecology and evolution of MHC. Specifically, our results lead to the conclusion that considering the population level alone is not sufficient to understand parasite-mediated selection. Even the across-host positive correlation between MHC allele richness and parasite richness demonstrated in earlier studies [11] , [12] gives only a narrow picture of the complex evolutionary process. Instead, the ecological pattern in which host–parasite interactions are organized is crucial to understand adaptive evolution of MHC. It is evident from our data that the direct and indirect effects hosts and parasites exert on each other are correlated with more than half of the variability in MHC diversity resulting from parasite-mediated selection. Yet, some parasite–supertype associations were not affected by the host–parasite network structure, indicating that associations can also depend solely on the parasite and supertype. This can happen, for example, when a parasite is specific to a host that has low MHC diversity resulting in independence from other host–parasite interactions. We note that because the parasite–supertype association network is probabilistic in nature, devising a clear-cut criterion or threshold for what is a ‘biologically meaningful’ parasite–supertype association may not be the best practice, and should also greatly depend on the research question and system. In fact, because this is a result of two interconnected networks ( Fig. 1 ), all associations are ‘meaningful’ to some extent because they all mutually affect each other. This reflects well the true biological complexity in interactions between parasites and supertypes mediated through hosts. Parasite–supertype association networks created for other communities may have other properties than those of the network described here, and this is a rich area for future research. Nature is dominated by complex dynamics between species co-evolution and the structure of the networks they assemble [28] . Here, host–parasite co-evolution is also dependent on MHC. Hosts that evolve resistance remove interactions from the host–parasite network (or weaken existing ones) and parasites that evolve new pathways of infection add interactions to the host–parasite network (or strengthen existing ones) through genetic change in MHC alleles. When such dynamics occur at the community level, they can simultaneously affect multiple hosts, parasites, MHC alleles and the interactions among them. For example, an overall reduction in the genetic resistance in a host population to a parasite owing to changes in allele frequencies will cause an increase in the parasites’ prevalence in the host population. If the parasite is not a strict host specialist, then selection imposed by the parasite on individuals of a second host species may also increase, thereby promoting MHC diversity in that host. This process can be extended to multiple hosts and parasites, eventually resulting in a complex network of indirect effects between hosts, parasites and MHC supertypes, whereby parasite-mediated selection on MHC supertypes of one or few hosts can have cascading effects on the MHC diversity of the whole host community. Hence, and following previous evidence that genetic diversity can shape community structure [29] , we propose to extend current hypotheses explaining mechanisms of parasite-mediated selection [9] to include multiple host–parasite interactions. For instance, according to the ‘rare-allele advantage hypothesis’ [9] , rare alleles in the host population confer better resistance than more frequent alleles because parasites have not had the time to evolve avoiding mechanisms (resistance). The rise of such an allele in a particular host species would weaken the host–parasite interaction in the network, with cascading effects on other species. With time, the rare allele becomes more frequent in the population and thus its selective advantage decreases as parasites evolve resistance. This would strengthen the host–parasite interaction, again affecting other species in the community. Once the allele becomes rare again, parasite adaptation for it also decreases, causing the selective advantage of the allele to increase again. Because changes to one interaction in the network have cascading effects on other interactions, there should be a dynamical interplay between the structural patterns of the host–parasite and host–supertype networks eventually affecting the co-evolution between parasites and MHC. This view is supported by the predictable nested pattern of parasite–supertype associations and by the modular network structure that indicates high co-evolutionary potential between particular parasites and supertypes. The association between host–parasite network structure and the diversity of MHC supertypes suggests that a perturbation to the structure of the host–parasite network may result in a concomitant perturbation to the host–supertype network. Human-driven environmental changes can alter the interactions between hosts and parasites [30] . For example, rodents and their associated parasites can invade disturbed areas, possibly creating new interactions between local rodents and invading parasites [31] . Such alteration to the host–parasite network may have consequences to the selection pressure imposed by parasites and to the evolution of MHC supertypes through indirect cascading effects. Because rodents are carriers of zoonotic parasites and pathogens [32] , [33] ( Supplementary Table 3 ), the ecological-evolutionary dynamics between altered host–parasite interactions and MHC may have implications for risk of zoonotic diseases [34] . Indeed, the rapid evolutionary potential of both hosts and parasites [34] makes genetic change possible even on ecological timescales. This study is the first to integrate tools and theory of network ecology with immunogenetics, providing novel insights into the evolution of functional MHC alleles in the context of community ecology. In particular, our results lead us to conclude that more than half of the variability in MHC diversity may be shaped by host–parasite interactions in the community, with reciprocal effects of the changes in MHC diversity on host–parasite interactions. This scales our view of MHC diversity from the population level to the community level. The complexity inherent to this model of network-based parasite-mediated selection promotes MHC diversity through indirect pathways, and suggests that the structure of host-parasite interactions plays a major role in the evolution of host immunity at the community level. Ethics statement All work with animals was approved by the French National Research Agency, project ANR 07 BDIV 012. Animals were treated in accordance with the guidelines of the American Society of Mammalogists and with the European Union legislation (Directive 86/609/EEC). None of the rodent species investigated were on the Convention on International Trade in Endangered Species of Wild Fauna and Flora (CITES) list or on the Red List of the International Union for Conservation of Nature (IUCN). Each trapping session was validated by the national, regional and local health authorities, and under an oral agreement of local land owners. Approval notices for trapping and investigating rodents were given by the Ethical Committee of Mahidol University, Bangkok, Thailand, number 0517.1116/661 and by the Ministry of Health Council of Medical Sciences, National Ethics Committee for Health Research Lao PDR, number 51/NECHR based on the validation of the rodents trapping book protocols of CERoPath [16] . Cambodia has no ethics committee overseeing animal experimentation. In addition, regional approval was obtained from the regional Head of Veterinary Service (Hérault, France) for sampling and killing rodents and harvesting rodent tissues (approval no. B 34-169-1). MHC genotyping Since previous studies have shown an association between helminthic infections and certain MHC alleles [5] , [7] , [35] , [36] , each individual in the data set ( Supplementary Data 1 ) was genotyped using a portion of the MHC class II DRB exon-2 functional gene that recognizes extracellular parasites such as helminths, by two independent runs of 454 GS-FLX sequencing following the procedure detailed in ref. 18 . In brief, the locus was amplified by PCR using a modified version of the primers JS1 (5′-GCCTCCCTCGCGCCATCAG-3′) and JS2 (5′-GCCTTGCCAGCCCGCTCAG-3′), which amplify a 171-bp fragment (excluding primers) of exon 2 from the DRB gene in several mammal species. These primers include in the 5′ position an individual-specific multiplex identifiers and the 454 adaptors required for the emulsion PCR and the 454 GS-FLX sequencing [18] . The SEquence Sorter & AMplicon Explorer software (SESAME ver 1.1B; ref. 37 ) was used to sort the sequences (that is, individual assignment of the sequences and removal of artefactual variants generated during PCR, emulsion PCR and 454 sequencing), and to determine the genotype of each individual. Gene duplication is common in MHC genes, and, in theory, an individual can have more than two alleles. However, this was ruled out for all the 11 species studied [18] . Thus, individuals of the rodent species used here had a maximum of two alleles amplified by the PCR primers. Supertype clustering The validated MHC alleles were clustered with similar antigen binding into supertypes as proposed in ref. 22 . The clustering to supertypes was based on 22 amino-acid sites detected as antigen-binding site on the basis of X-ray data of peptide class II protein complexes [38] , [39] and/or detected under positive selection using the HyPhy programme [40] included in the MEGA5 software [41] . Each of the 22 amino acids forming the antigen-binding site was characterized by five physicochemical descriptor variables: z1 (hydrophobicity), z2 (steric bulk), z3 (polarity), z4 and z5 (electronic effects). Our final matrix for supertype classification had 276 rows representing unique alleles and 110 columns (5 physicochemical descriptors for 22 sites). We clustered the unique alleles into supertypes using a K -means clustering algorithm and model selection following the procedure described in ref. 23 with the function ‘find.clusters’ from package ‘adegenet’ (version 1.3-9; ref. 42 ). In brief, the optimal number of supertypes (clusters) is defined as the minimal number of clusters after which the Bayesian Information Criteria (BIC) decreases by a negligible amount as indicated by the curve of BIC values as a function of cluster number ( Supplementary Fig. 2 ). We used a manual classification criterion as recommended in the ‘adegenet’ package reference. However, classification is a stochastic process (that is, there is no absolute true classification) and we thus validated our classification as follows. We ran 500 automated classifications using the option ‘smoothNgoesup’, in which the selected number of clusters is the K after which increasing the number of clusters leads to increasing the BIC in a loess-smoothed curve. Our manual classification to 24 supertypes was almost identical to the mean of the automated classification process and fell within its 95% confidence intervals (CIs; mean±s.d. 23.23±3.7; 95% CI (16,29)). Furthermore, we used a measure of normalized mutual information [43] , based on information theory, to examine the differences between the automated and manual classifications in terms of allele identities. The index quantifies the amount of certainty that we can have in our manual classification by observing an automated one. If the manual classification is identical to the automated one (clusters in the manual and automated classifications contain the exact same alleles), the index takes its maximum value of 1. If the classifications are totally independent (complete mismatch in clustering), its value is 0 (see details in ref. 43 ). The average mutual information across the 500 automatic classifications was 0.85, indicating that our classification was accurate. In Loei, a classification of the 144 alleles found across individuals revealed 18 supertypes, one of which was not harboured by infected individuals and was omitted from analyses. Our manual classification to supertypes was almost identical to the mean of the automated classification and fell within its 95% CIs (mean±s.d. 18.28±2.4; 95% CI (12,21)). The average normalized mutual information across the 500 automatic classifications was 0.88, indicating that our classification was accurate. Furthermore, a comparison of supertype classification between Loei and the pooled data set resulted in a normalized mutual information of 0.84. This essentially indicated that by knowing the classification in the Loei data set, we can know the classification in the pooled data set and vice versa with 84% certainty, indicating a great overlap in the classification of alleles to particular supertypes even between the data sets. We matched the two alleles of an individual with their corresponding supertypes such that each individual in the data set was also characterized by a pair of supertypes. To simplify, in this study, the terms genotype, homozygote and heterozygote refer to supertypes, not alleles, and are defined as follows. A supertype is a functional group to which an allele belongs, and a genotype is a combination of two supertypes (in case of a heterozygote) or one supertype (in case of a homozygote) to which the two alleles of an individual belong. For example, if alleles A and B were classified as supertype no. 1, and allele C was classified as supertype no. 2, an individual bearing alleles A and B would be a homozygote with a genotype 1-1, whereas an individual bearing alleles B and C would be a heterozygote with a genotype 1-2. At the individual host level, susceptibility to helminths can result from one of the two alleles or from a co-dominant effect of both, also depending on the parasite in question [13] . It is common in studies of MHC diversity to use only alleles/supertypes, rather than genotypes in statistical analyses [5] , [6] , [44] . However, owing to the lack of knowledge of the genetic mechanism, and because working with genotypes would create sparse networks, we used supertypes and validated our analyses with genotypes [13] . The results were qualitatively similar and we thus present only analyses done with supertypes. Analyses done using genotypes can be found in Supplementary Methods . Phylogeny We built a phylogenetic tree based on molecular data of the cytochrome b mitochondrial gene. We compiled cytochrome b sequences from the NCBI gene bank and used a maximum likelihood analysis with the GTR+G+I substitution model of molecular evolution with the aid of the function ‘phymltest’ in the R package ‘ape’ [45] . To ensure that our results were not affected by the way we constructed the tree, we re-ran our analyses with two other trees from refs 46 , 47 , which did not change our results qualitatively ( Supplementary Methods ). Similarity analysis In the host–parasite ‘ecological’ network, we connected between a rodent species and a helminth when at least one rodent individual was infected by this helminth. Interaction weights (matrix cell values in Fig. 2a ) were set as parasite prevalence—the fraction of individuals of a given rodent species infected by a given helminth. We described the diversity of supertypes across hosts with an ‘immunogenetic’ network ( Fig. 1 ). We connected a supertype and a host if at least one infected individual of the host harboured the supertype. The weights of network interactions (matrix cell values in Fig. 2b ) were determined as supertype frequency—the number of infected individuals of a given rodent with a given supertype, divided by the total number of individuals of that host harbouring the supertype. In calculating interaction weights, heterozygote individuals were counted twice (once for each of their supertypes), whereas homozygote individuals were counted once. This assured that interaction weights represented supertype frequencies rather than individual frequencies. We examined whether hosts infected by similar parasites with a similar prevalence harbour similar MHC supertypes with similar frequencies, while controlling for phylogenetic effects, using a partial Mantel’s test following ref. 24 . For this, we created dissimilarity matrices for the host–parasite and host–supertype networks (matrices) using the Ružička index (RI), implemented in the R package ‘vegan’ [48] , defined as: RI=2 D /(1+ D ), where D is dissimilarity between hosts j and k given by D jk =Σ |(x mj −x mk )|/Σ (x mj + x mk ), within which x m is the prevalence of parasite m (or frequency of supertype m ) on hosts j and k , summed for all parasites infecting (or supertypes harboured by) j or k . The RI is a quantitative version of the Jaccard index and allows for direct comparisons between hosts [49] , [50] . An RI value of 1 indicates maximum dissimilarity, where no parasites (or supertypes) are shared between a pair of hosts, whereas an RI value of 0 indicates that parasites infect (or supertypes are harboured by) hosts with a similar prevalence (frequency). To disentangle the effect of neutral species traits (or genes), which are assumed to be described by phylogeny, from that of parasite-mediated selection on MHC diversity, we created a phylogenetic distance matrix between pairs of host species using the function ‘cophenetic.phylo’ (R package ‘ape’, version 3.0-7), which calculates the sum of the length of the branches between pairs of species. We used this matrix as a control matrix in the partial Mantel’s test, which examines the null hypothesis of no relationship between parasite diversity and MHC diversity using dissimilarity matrices. If host–parasite network structure is correlated with diversity of MHC supertypes across hosts (host–supertype network structure), we expect a positive and significant correlation between the host–parasite and host–supertype dissimilarity matrices ( Supplementary Fig. 3 ). Bayesian analysis We calculated a matrix of parasite–supertype probabilistic associations, M obs , by representing our system as a simple Bayesian network with three random variables (nodes): host, parasite and supertype ( Fig. 3 ). For this Bayesian network, we recalculated the host–parasite and host–supertype matrices to create two conditional probability tables (rows sum to 1) representing the probability of sampling a parasite p j or a supertype s k given a host h i . That is, the number of individuals of h i infected with p j divided by the total number of infected individuals of h i (ecological matrix) and the number of infected individuals of h i harbouring s k divided by the total number of infected individuals of h i (immunogenetic matrix). Biologically, the matrices represent the strength of infection of a parasite p j on host h i in comparison with all other parasites and the level of susceptibility/resistance conferred by a supertype s k for a given host h i in comparison with all other supertypes. The analysis also requires a conditional probability table for the host node of the Bayesian network. Because we did not have any preference for selecting a particular host, we assumed a uniform distribution for the probability of obtaining a host, P( h i )=1/11 (total of 11 hosts). Given the Bayesian network and the conditional probability tables, we used the chain rule of Bayesian networks and Bayes theorem (see Proof 1 and equation (4)) to calculate the values of the matrix M obs , depicting the probability of obtaining a supertype s k given a parasite p j across hosts ( Fig. 3 ). Proof 1: To examine whether the parasite–supertype associations (cell values of M obs ) are correlated with the structure of the host–parasite network, we compared them with those derived from 1,000 matrices recalculated after randomizing the ecological matrix using two null models. The first null model, based on the IA algorithm from ref. 51 , reshuffles only the values of the host–parasite network. The algorithm reassigns individuals randomly to matrix cells with probabilities proportional to observed row and column abundance totals until the matrix-wide total number of individuals is reached. The structure is not altered (that is, zero cells are kept the same in the randomized matrices). Therefore, non-observed host–parasite interactions are regarded to as ‘forbidden’. The second algorithm reshuffles both the values and structure of the host–parasite matrix and is a modified version of the IF algorithm from ref. 51 . This algorithm first shuffles the matrix according to the swap algorithm for binary matrices [26] and then assigns individuals randomly to matrix cells as in the previously described algorithm. In this case, non-observed host–parasite interactions are not regarded to as forbidden and are allowed to occur in the random matrices. We determined statistical significance (at the α =0.05 level) as the proportion of association probabilities obtained by random that were either equal or larger or equal or lower than the observed association probabilities. Forbidden interactions were excluded from this calculation ( Supplementary Fig. 5 ). We used a two-tailed permutation test because random probabilities of parasite–supertype associations could be either higher or lower than the observed probability. When calculating the proportion of significant interactions in the model that shuffles only interaction values, we omitted 60 parasite–supertype associations (11% of the total 520) that involved parasites that infect a single host species because the distribution of parasite–supertype associations resulting from the null model for such parasites consisted of a single value, always resulting in a significant parasite–supertype association. We note that both our null models were very conservative in the sense that they present elevated chances of not finding a significant pattern where it really does exist, as compared with models with less strict rules for network randomization [26] . Nestedness and modularity We calculated nestedness using the NODF index [27] implemented in the software Aninhando [52] . We calculated modularity using the QuanBiMod algorithm for quantitative bipartite networks [53] as implemented in the package ‘bipartite’ (version 2.03; ref. 54 ) in R using default values. To examine whether modules of supertypes and parasites were indeed the result of an evolutionary process rather than a random one, we explored whether our network was significantly more modular than random networks obtained by using both null models as described above (1,000 random networks per null model) using a one-tailed permutation test because random networks are expected to have lower modularity than the observed network. Parasite specificity We used the Paired Differences Index [55] as a quantitative measure of parasite specificity for hosts (in the host–parasite network) or supertypes (in the parasite–supertype network). The index contrasts the strongest interaction of a parasite on a host (or the strongest association of a parasite with a supertype), with the remaining interactions with other hosts (or remaining associations with other supertypes). We used the normalized version of the index, which divides the index for each species by the maximum of interactions. Thereby, parasite species can be compared among each other and values range between 0 (perfect generalist) and 1 (perfect specialist). We calculated the index using the function ‘PDI’ in the R package ‘bipartite’. Data and R code The data and R code used in the analyses and to construct Figs 2 and 3 and Supplementary Tables and Figures are available as Supplementary Methods and Supplementary Data 2 , Supplementary Data 3 , Supplementary Data 4 , Supplementary Data 5 . The multiplexed raw sequences (.fasta files and .qual files) and the validated sequences of the 276 alleles are available from the Dryad Digital Repository: http://doi.org/10.5061/dryad.mq7n0/1 . Accession codes: The demultiplexed raw sequences generated in this study have been deposited in NCBI Short Read Archive (SRA) under the accession code SRP047116 . How to cite this article: Pilosof, S. et al. Host–parasite network structure is associated with community-level immunogenetic diversity. Nat. Commun. 5:5172 doi: 10.1038/ncomms6172 (2014).